Spectroscopic observation of iodosylarene metalloporphyrin adducts and manganese(V)-oxo porphyrin species in a cytochrome P450 analogue Different metalloporphyrin model compounds have been synthesized to study the mechanisms of cytochrome P450s with various terminal oxidants, and numerous intermediates have been reported. However, the detailed mechanism of the oxygen atom transfer from iodosylarene to the substrates remains unclear. Here we report the direct ultraviolet-visible spectroscopic observation of the soluble iodosylarene-manganese porphyrin adduct following catalytic oxidation using 2,4,6-tri- tert -butylphenol as the reductant. When the reductant is changed to cis -stilbene, the rate-determining step also changes. Both the iodosylarene-manganese porphyrin adduct and [(porphyrin)Mn(V)=O] species may be simultaneously observed. In the absence of reductant, the adduct of iodosylarene with sterically hindered [Mn(meso-tetrakis(2,6-dichlorophenyl)porphinato)Cl] is immediately formed, and smoothly converted into a high-valent [(porpyrinato)Mn=O]. Electrospray ionization mass spectrometry analysis of the reaction further confirms the transformation between these species. This study provides an insight into the mechanism of oxygen transfer within the haem-containing enzymatic systems. For more than 30 years the study of cytochrome P450 has been at the frontier of research [1] , [2] . It exhibits promising catalytic behaviour for a host of oxidative reactions, and so a primary goal of cytochrome P450 research is in the application of these enzymes, or their derivatives, in catalytic oxidation of unactivated C-H bonds, such as the hydroxylation of cyclohexane. Many synthetic metalloporphyrin model compounds have been synthesized to probe the mechanisms of the behaviours of cytochrome P450 oxygenases [3] , [4] , [5] , [6] , [7] , [8] , [9] , [10] , [11] , [12] , [13] , but the detailed pathways are still elusive, especially for the steps involving highly reactive intermediates. For a long time, it has been believed that oxoiron (IV) porphyrin π-cation radical (named as Compound I) is the unique reactive intermediate in cytochrome P450 catalysed oxidative reactions ( Fig. 1c ) [14] . Spectra of the active species were obtained from stopped-flow reaction using global analysis techniques by Egawa and Sligar [15] , [16] , [17] . Recently, Green and co-workers [18] , [19] reported an elegant characterization of the cytochrome P450 Compoud I. However, along with the accumulation of various evidence, multiple oxidizing species ( Fig. 1a ) were speculated to be able to transfer oxygen atoms to the substrates [20] , [21] , [22] and the mechanisms were found to be more complicated than those initially proposed [23] , [24] . For example, ferric-peroxo species were proven to react with electrophiles [25] . In addition, a number of oxidant-metalloporphyrin adducts [26] , [27] , [28] and oxidant-nonheme adducts [29] , [30] , [31] , which have been speculated without direct spectroscopic evidence during the catalytic process, might directly react with substrates instead of the formation of metal-oxo intermediates. 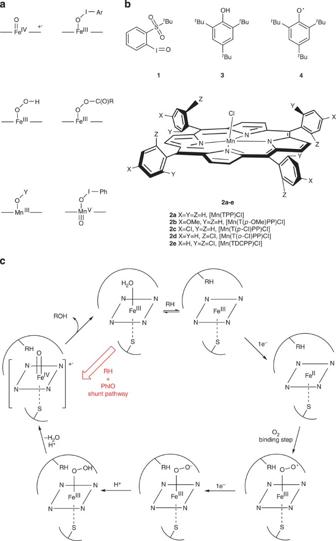Figure 1: Schematic illustrations. (a) Possible reactive intermediates. (b) Structure of substrates and catalysts used in this work. (c) Oxidative catalytic cycle of cytochrome P450. Figure 1: Schematic illustrations. ( a ) Possible reactive intermediates. ( b ) Structure of substrates and catalysts used in this work. ( c ) Oxidative catalytic cycle of cytochrome P450. Full size image Peroxyacids [26] , [32] , [33] , [34] , [35] , hydroperoxides [36] , [37] , [38] , [39] or inorganic salts [40] , [41] , [42] , [43] , [44] , [45] were generally employed as terminal oxidants in mechanistic studies, and the reactions were always performed in water or mixed solvents (such as CH 3 OH/H 2 O or CH 3 CN/H 2 O). In fact, PhIO is often mechanistically cleaner than these alternatives [46] . For example, the reaction between iodosylbenzene and [Mn(TPP)Cl] (TPP=meso-tetraphenylporphinato dianion, see Fig. 1b , compound 2a ) is considered to be a closer model of P450 than that of alkyl hydroperoxide and [Mn(TPP)Cl] [47] . But the detailed mechanism regarding the oxygen transfer from PhIO to substrates is still unclear owing to the lack of kinetic and spectral data in live catalytic processes. This dilemma is because of the insolubility of PhIO, which results from the polymeric structure derived from the intermolecular I-O bond [48] , [49] . To gain further insights into the mechanism, soluble ArIO is required. Recently, Protasiewicz and co-workers [50] synthesized the soluble iodosylbenzene derivative ArIO ( Fig. 1b , compound 1 ) by introducing an intramolecular I-O bond to avoid the formation of polymeric structure. Later, Collman et al. [51] used this kind of iodosylarene in kinetic investigations of olefin epoxidation, using manganese(III) porphyrin as the catalyst. Therefore, the soluble iodosylarene derivative enables us to observe intermediates by ultraviolet–vis spectroscopy and obtain kinetic data. Herein, we investigate the kinetic behaviours in catalytic reactions by various metalloporphyrins with soluble iodosylarene as the terminal oxidant in organic solvent. We also report the direct observations of Mn(V)-oxo and the oxidant-metalloporphyrin adduct in ultraviolet–vis spectra for the first time. On the basis of kinetic data, obtained by ultraviolet–vis spectroscopy and electrospray ionization mass spectrometry (ESI-MS) analysis, a detailed mechanism is proposed, which indicates that the ‘shunt pathway’ [2] may not be one step but a more complicated process including the formation of a ArIO-metalloporphyrin adduct followed by the heterolysis of I-O bond to form the highly reactive metal-oxo intermediate. Rapid high valent intermediate trapping reactions The reaction between TBPH (2,4,6-tri- tert -butylphenol) and ArIO in the presence of manganese porphyrin was initially investigated. By presenting a stable phenoxy radical the TBPH was able to trap a high valent intermediate [32] . 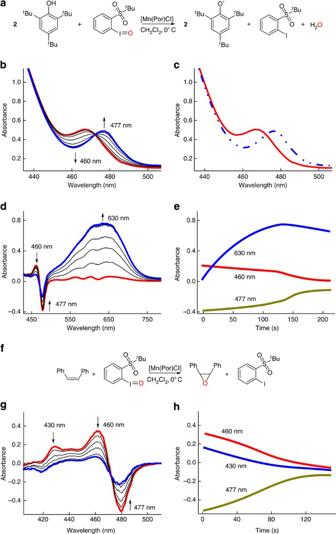Figure 2: Ultraviolet–vis spectra of the catalytic oxidative reactions. (a) Catalytic reaction of TBPH. (b) Time slices are from 0 to 30 s, one spectrum per 6 s. (c) Red line: obtained spectrum. Blue line: the spectrum of [Mn(TPP)Cl] combined with TBPH. (d) [TBPH], [ArIO] and [Cat]=1.25 × 10−2, 2.5 × 10−3and 6.25 × 10−6M, respectively. This figure shows the spectra at 0, 25, 50, 75, 100 and 125 s. (e) Red: 460 nm, dark yellow: 477 nm, blue: 630 nm. (f) Catalytic oxidation ofcis-stilbene. (g) This figure shows the spectra at 0, 5, 10, 15, 20 and 25 s. (h) Blue: 430 nm, red: 460 nm, dark yellow: 477 nm. Figure 2b shows the spectrum for the first 30 s after the addition of catalyst [Mn(TPP)Cl] into a CH 2 Cl 2 solution of TBPH and ArIO ([TBPH]: [ArIO]: [Mn(TPP)Cl]=1500: 75: 1). The colour of the solution gradually changed from yellow to blue along with rapid increasing peaks at 399 and 630 nm, which were assigned as the characteristic absorbance of the 2,4,6-tri- tert -butylphenoxy (TBP) free radical 4 . Additionally, [Mn(TPP)Cl] ( λ max =477 nm) disappeared at the beginning of the reaction, while a new species with an absorbance at 460 nm was formed ( Fig. 2c , red line). In order to obtain clearer spectral information about the changes of the catalyst during this transformation, a mixture of 2a and 3 was set as the background and the spectrum was collected after the addition of 1 . Consequently, the peak at 477 nm, corresponding to 2a , rapidly decreased, quickly reaching below baseline (a reversal peak in Fig. 2d ). The peak then gradually increased back to near zero by the time that the oxidant was consumed. Meanwhile, the peak at 460 nm reached to its maximum at the beginning and then decreased to zero after the completion of the reaction (for information about changes the catalyst imposes in Fig. 2d see Supplementary Fig. S15 ). Figure 2: Ultraviolet–vis spectra of the catalytic oxidative reactions. ( a ) Catalytic reaction of TBPH. ( b ) Time slices are from 0 to 30 s, one spectrum per 6 s. ( c ) Red line: obtained spectrum. Blue line: the spectrum of [Mn(TPP)Cl] combined with TBPH. ( d ) [TBPH], [ArIO] and [Cat]=1.25 × 10 −2 , 2.5 × 10 −3 and 6.25 × 10 −6 M, respectively. This figure shows the spectra at 0, 25, 50, 75, 100 and 125 s. ( e ) Red: 460 nm, dark yellow: 477 nm, blue: 630 nm. ( f ) Catalytic oxidation of cis -stilbene. ( g ) This figure shows the spectra at 0, 5, 10, 15, 20 and 25 s. ( h ) Blue: 430 nm, red: 460 nm, dark yellow: 477 nm. Full size image Figure 2e indicates the relationship between the observed species during the reaction process. During the first 10 s, the product TBP free radical 4 was accumulated quickly while the concentration of the new species at 460 nm was unchanged. When the oxidant was being gradually consumed, the rate of formation of 4 notably decreased while the intermediate transformed back to 2a . Catalytic olefin epoxidation reaction When cis -stilbene was employed as the reductant instead of TBPH, completely different reaction spectra were observed, shown in Fig. 2g . The mixture of cis -stilbene and [Mn(TPP)Cl] 2a in CH 2 Cl 2 was set as the reaction background for the ultraviolet–vis studies. After iodosylarene was added, the peak at 477 nm, which represented the absorbance of [Mn(TPP)Cl], quickly maximized below the baseline and then moved back to near zero at the end of the reaction (the reversal peaks in Fig. 2g ). Two peaks at 430 and 460 nm were observed simultaneously and then decayed ( Fig. 2g ). Gas chromatography (GC) analysis showed a cis -stilbene epoxide yield of 31% with respect to the amount of ArIO initially used. The relationship among the observed species during the reaction period is shown in Fig. 2h . The new absorbance at 430 nm indicated another new observable species in the catalytic reaction. Kinetic data The kinetic investigation of the catalytic rapid free radical trapping reaction was then performed at 0 °C in CH 2 Cl 2 using quick-mixing method through a stopped-flow or ultraviolet–vis spectrometer. The results in Fig. 3a show an increase in reaction rate when a higher concentration of soluble ArIO 1 was employed. By plotting the initial rates versus the concentration of 1 , first-order dependence of the catalytic reaction on the oxidant ArIO 1 was revealed ( Fig. 3b ). Changing the concentration of TBPH has no effect on the reaction rate ( Fig. 3c ). Plotting the concentration of TBPH and the catalytic reaction rates, shown in Fig. 3d , suggested that the catalytic reaction rate was independent on the reductant TBPH 3 . Besides, the catalytic reaction also showed a first-order kinetic dependence with respect to the Mn catalyst ( Supplementary Fig. S9 ). Similar kinetic results were obtained when other catalysts were used ( Supplementary Figs S1–S8 ). Moreover, an identical reaction order was obtained when the reaction was performed at −10 °C ( Supplementary Figs S10–S11 ). 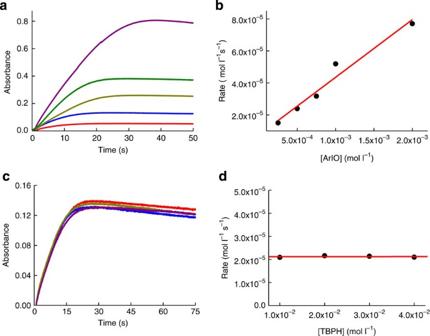Figure 3: Kinetic data. Time interval=50 ms.yAxis ofFig. 3aandFig. 3crepresent the absorbance at 630 nm. (a) [TBPH] and [Mn(TPP)Cl] were 2 × 10−2and 6.7 × 10−6M, respectively. [ArIO] was 2.5 × 10−4, 5 × 10−4, 7.5 × 10−4, 1 × 10−3and 1.5 × 10−3M, respectively. (b) First-order dependence on [ArIO]. (c) [ArIO] and [Mn(TPP)Cl] were 5 × 10−4and 6.7 × 10−6, respectively. [TBPH] was 1 × 10−2, 2 × 10−2, 3 × 10−2and 4 × 10−2M, respectively. (d) Zero-order dependence on [TBPH]. Figure 3: Kinetic data. Time interval=50 ms. y Axis of Fig. 3a and Fig. 3c represent the absorbance at 630 nm. ( a ) [TBPH] and [Mn(TPP)Cl] were 2 × 10 −2 and 6.7 × 10 −6 M, respectively. [ArIO] was 2.5 × 10 −4 , 5 × 10 −4 , 7.5 × 10 −4 , 1 × 10 −3 and 1.5 × 10 −3 M, respectively. ( b ) First-order dependence on [ArIO]. ( c ) [ArIO] and [Mn(TPP)Cl] were 5 × 10 −4 and 6.7 × 10 −6 , respectively. [TBPH] was 1 × 10 −2 , 2 × 10 −2 , 3 × 10 −2 and 4 × 10 −2 M, respectively. ( d ) Zero-order dependence on [TBPH]. Full size image Reactions between ArIO and manganese porphyrins Reactions between Mn-porphyrins and soluble iodosylarene, in the absence of a reductant, were investigated. [Mn(TDCPP)Cl] 2e (6.25 × 10 −6 M) in CH 2 Cl 2 at 0 °C was set as the background of the in situ ultraviolet–vis experiment (TDCPP=meso-tetrakis(2,6-dichlorophenyl)porphinato dianion). After the oxidant ArIO 1 (2.5 × 10 −3 M) was added, the peak at 477 nm quickly reached the maximum absorbance below baseline (red line in Fig. 4a ). Meanwhile, two new peaks at 460 and 422 nm were detected (red line in Fig. 4a ). Then, the peak at 460 nm decreased and the peak at 422 nm increased simultaneously ( Fig. 4a ). Two minutes later, the reductant 3 (3.8 × 10 −2 M) was added to this mixed solution. The catalytic reaction of 1 with 3 immediately took place, and the concentration of the TBP free radical increased with time (the wine line in Fig. 4b ). When catalyst 2d was employed in the reaction, similar phenomena were observed. 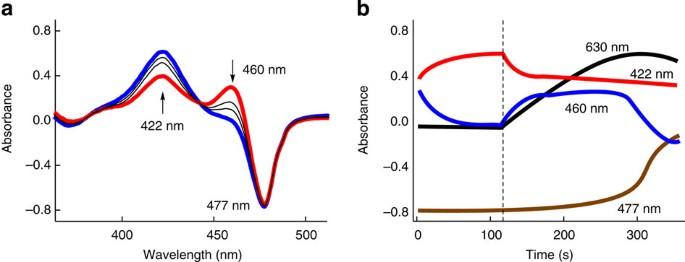Figure 4: Studies ofin situreactions. (a) Reaction between ArIO and [Mn(TDCPP)Cl]. (b) TBPH was added to the mixture 2 minutes later after the combination of catalyst and ArIO. [TBPH]=3.8 × 10−2M. This figure shows the relationship between the observed species. TBPH was added at 120 s. Red: 422 nm, blue: 460 nm, dark yellow: 477 nm, wine: 630 nm. Figure 4: Studies of in situ reactions. ( a ) Reaction between ArIO and [Mn(TDCPP)Cl]. ( b ) TBPH was added to the mixture 2 minutes later after the combination of catalyst and ArIO. [TBPH]=3.8 × 10 −2 M. This figure shows the relationship between the observed species. TBPH was added at 120 s. Red: 422 nm, blue: 460 nm, dark yellow: 477 nm, wine: 630 nm. Full size image When the less hindered catalyst [Mn(TPP)Cl] 2a was used in this study, the peak at 460 nm was observed as was the peak at 430 nm. However, these two peaks rapidly decreased in the absence of a reductant. Although TBPH 3 was added after 3 min, nearly no TBP free radical was formed, and no 2a was regenerated ( Supplementary Figs S12–S14 ). The decrease in the peak at 460 nm was owing to its transformation into the species at 430 nm while the decrease of 430 nm was owing to the destruction of the metalloporphyrin structure in the presence of excess oxidant [52] . When less hindered Mn-Porphyrins catalysts 2b , and 2c were employed, similar phenomena were observed. Reaction between ArI and the active intermediate (422 nm) Three equivalent of ArIO was added into the CH 2 Cl 2 solution of [Mn(TDCPP)Cl] at 0 °C in the absence of a reductant. Similar to the above result, the intermediate at 422 nm was formed and this peak remained unchanged for several minutes under these conditions. When [Mn(TDCPP)Cl] completely transformed into the intermediate at 422 nm, excess ArI was added to this solution. The peak at 422 nm gradually disappeared while the peak at 477 nm increased ( Fig. 5a ). In addition, the peak at 460 nm appeared at the very beginning and then disappeared. Fig. 5b shows the relationship of these three peaks during the reaction process. 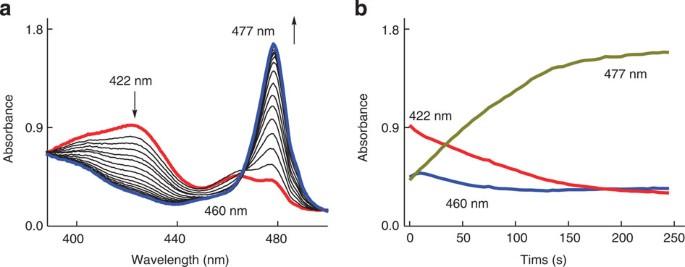Figure 5: Reaction between ArI and the intermediate (422 nm). (a) ArI was added to the intermediate. (b) Relationship between the observed species. Red: 422 nm, blue: 460 nm, dark yellow: 477 nm. Figure 5: Reaction between ArI and the intermediate (422 nm). ( a ) ArI was added to the intermediate. ( b ) Relationship between the observed species. Red: 422 nm, blue: 460 nm, dark yellow: 477 nm. Full size image First-order kinetics with respect to the oxidant ArIO 1 and zero-order kinetic with respect to the concentration of reductant TBPH 3 have been determined in the reaction of soluble ArIO with TBPH in the presence of Mn-porphyrin 2a . Weak non-covalent interactions between Mn(IV) oxo complex and the substrates resulted in formation of an encounter complex intermediate, as recently reported in C-H hydrogen atom transfer reactions. [53] Independence with respect to the substrate was observed when the saturated concentration was reached if the decomposition of this intermediate was the rate-determining step. However, this saturated kinetic could be ruled out in this work by the following reasons: (1) if the decomposition of the encounter complex was rate-determining step, it was supposed to show zero-order dependence on ArIO while first-order dependence was obtained in our investigation; (2) high-valent metal-oxo porphyrin species was generally considered to be much more active than non-haem metal-oxo species [29] and TBPH was easily abstracted to form a relatively stable free radical, so this encounter complex could not be formed under this condition. Therefore, as well-established mechanism, one could believe that Mn(V)-oxo should be one of the reaction intermediates, and TBPH would react with this active species to generate the free radical. Thus, the above experimental results indicated that the reaction between Mn(V)-oxo and TBPH is fast, and Mn(V)-oxo should not be involved in the rate-determining step. As a result, the accumulation of Mn(V)-oxo species could not be observed during the ‘live’ catalysis process. If the Mn(V)-oxo species was formed directly from [Mn(TPP)Cl] 2a in one step, 2a should be the resting-species of the Mn catalyst. During the ‘live’ catalytic period, one should be able to observe a spectrum shown in Fig. 2c in blue. In that case, the peak at 477 nm ([Mn(TPP)Cl] 2a ) should maintain unchanged in the overall reaction. However, a new peak at 460 nm appeared in our gained spectra. Moreover, from Fig. 2e , it could be observed that the species with λ max at 460 nm was the resting-species in the first 10 s of the catalytic reaction. During this 10 s, the TBP free radical formation showed a pesudo-zero-order kinetic behaviour, which indicated that the period was under ‘live’ catalytic process. All of them together revealed that the real steady-state Mn catalyst was not [Mn(TPP)Cl] 2a , but the one with absorbance at 460 nm. Furthermore, it also indicated that the mechanism may be more complicated than the previously proposed. In metalloporphyrin catalysed alkenes epoxidation reactions, the rate-determining step has been determined to be the oxygen atom transfer from the high-valent metal-oxo to alkenes [41] . It indicates that the high-valent metal-oxo species is the steady-state, and should be able to be observed by ultraviolet–vis spectroscopies. By using the soluble ArIO 1 , the expoxidation of cis -stilbene was investigated. It was different from the reaction in which TBPH 3 was the reductant. Another intermediate (peak at 430 nm), was observed in the spectrum ( Fig. 2g ). The great change of the λ max (from 477 to 430 nm) indicated the change of the oxidation state of metal and known synthetic high-valent manganese-oxo porphyrins have λ max in the range of 420 to 450 nm [6] , [10] . In addition, Newcomb et al. [12] have reported that λ max of [(TPP)Mn(V)=O] was about 430 nm by using laser flash photolysis method. So this intermediate with its λ max at 430 nm might be [(TPP)Mn(V)=O]. Moreover, other possibilities of this species have been proposed, such as dinuclear complex [ClMn(TPP)(OIAr)] 2 O (420 nm) reported by Hill [5] or a mononuclear complex [Mn(TPP)(OAr)(OIAr)] (422 nm) reported by Shim [54] . For the dinuclear one, though it was also able to oxidize alkanes, no epoxidation of olefins was reported by using this species. [55] For the mononuclear one, it was found that a derivative of phenol or benzoic acid as the axial ligand was crucial for the formation of the mononuclear species. In addition, when catalyst 2e was added to the solution of another terminal oxidant NaClO, the same peak at 422 nm, which was shown in Fig. 4a when ArIO was used, can be obtained ( Supplementary Fig. S16 ). This observation indicated that the peak at 430 nm (for [Mn(TPP)Cl]) or 422 nm (for [Mn(TDCPP)Cl]) should be a metal-oxo species but not a metalloporphyrin-oxidant complex. Therefore, we assigned that this intermediate (peak at 430 nm) was probably [(TPP)Mn(V)=O]. The co-existence of the intermediate (peak at 460 nm) with [Mn(Por)(V)=O] (peak at 430 nm) might be due to an reversible equilibrium ( vide supra ). These experiments also indicated that the reaction might have more complicated kinetic behaviour. From the reported spectral data of Mn(V)=O porphyrin species and our obtained spectrum, a conclusion could then be made to put forward that the intermediate at 460 nm should not be Mn(V)=O porphyrin complex and the formation of metat-oxo species (shunt pathway) is supposed to include more than one step. Groves [3] had proposed an iodosylbenzene-manganese(III) porphyrin adduct in 1980. They considered that ArIO-metalloporphyrin adduct should be involved in epoxidations of olefins [4] . Besides, Collman also speculated the ArIO-metalloporphyrin adduct as a possible reactive intermediate in an iron porphyrin alkane hydroxylation system [56] . Recently, Nam had observed an equilibrium between iodosylbenzene-Iron porphyrin intermediates and oxoiron(IV) porphyrin π-cation radicals and the equilibrium favored the formation of ArIO-iron porphyrin intermediates when the porphyrin ligand was electron deficient [57] . They also found that the heterolysis rate of the I-O bond was relatively slower if aprotic solvent (such as CH 2 Cl 2 ) was used [28] . Based on the kinetic and spectroscopic evidences from the ‘live’ catalytic process previously discussed, we speculated that the intermediate with the absorbance around 460 nm was ArIO-manganese porphyrin adduct, and that the ‘shunt pathway’ involved two steps: the formation of an ArIO-metalloporphyrin adduct followed by the heterolysis of I-O bond to form the highly reactive metal-oxo intermediate, which is shown in Fig. 6 . 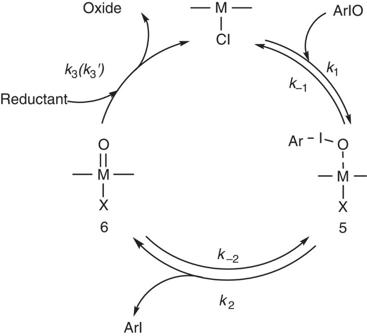Figure 6: Proposed mechanism. K1: rate constant of the formation of ArIO-manganeseporphyrin adduct. K2: rate constant of the formation of Mn(V)=O porphrin. K3(K3′): rate constant of the reaction between Mn(V)=O and TBPH (cis-stilbene). Figure 6: Proposed mechanism. K 1 : rate constant of the formation of ArIO-manganeseporphyrin adduct. K 2 : rate constant of the formation of Mn(V)=O porphrin. K 3 (K 3 ′): rate constant of the reaction between Mn(V)=O and TBPH ( cis -stilbene). Full size image As we speculated in Fig. 6 , when TBPH 3 was used as the reductant ( k 3 >> k 2 and k 1 >> k 2 ), the formation of [Mn(Por)(V)=O] intermediate 6 was the rate-determining step and the intermediate 5 was the steady-state of Mn catalyst, which we can observe in ultraviolet–vis spectrum. When cis -stilbene was employed as the reductant, the accumulation of 6 can be observed in ultraviolet–vis spectrum as the rate of the oxygen transfer from intermediate 6 to the olefin is much slower. Thus, the obtained spectrum can be well explained. Based on the speculation in Fig. 6 , we assigned that the species represented by the peak at 460 nm was the adduct of [Mn(TDCPP)Cl] 2e with ArIO 1 , and the other species represented by the peak at 422 nm was [(TDCPP)Mn(V)=O] intermediate. In the first 2 min in Fig. 4b , intermediate 5 (460 nm) completely converted to intermediate 6 (422 nm). Addition of TBPH would cause the free radical trapping reaction between metal-oxo species and TBPH. As the formation of intermediate 6 was the rate-determining step, the accumulation of intermediate 5 would be observed and the signal at 460 nm increased at the beginning of the formation of TBP free radical and then maintained unchanged during the catalytic process, which was very similar to the spectra shown in Fig. 2d and e . It is noteworthy that the adduct of [Mn(TDCPP)Cl] 2e with ArIO 1 represented by the peak in 460 nm was the steady-state Mn catalyst intermediate due to the following reasons: (1) the peak at 460 nm immediately increased as long as the reductant 3 was added, and it kept to be constant during the increasing of TBP free radical when it reached maximum (the blue line in Fig. 4b ); (2) the peak at 422 nm immediately decreased after the addition of 3 (the red line in Fig. 4b ); (3) when the oxidant 1 was completely consumed, the adduct (represented by 460 nm) was consumed, and 2e was regenerated (the dark yellow line in Fig. 4b ). In addition, the equilibrium between manganese porphyrin, adduct 5 and active intermediate 6 ( Fig. 6 ) was also coincident with the experimental results in Fig. 5 . When excess ArI was added to the solution of [(TDCPP)Mn(V)=O] intermediate, this species gradually transformed back to adduct 5 and finally the initial form of manganese porphyrin, so the peak at 477 nm would appear. This result was similar to the report of iron porphyrin by Nam [57] . In order to confirm the proposed mechanism, ESI-MS analysis of the reaction between manganese porphyrin and ArIO was performed. As shown in Fig. 7 , ArIO-metalloporphyrin adduct was formed at the very beginning of the reaction ( Fig. 7a and d ). For [Mn(TPP)Cl], a peak at m/z 1007 ([Mn(TPP)(ArIO)] + , MW 1007.84) appeared and then decayed along with the formation of another peak at m/z 683 ([Mn(O)(TPP)] + , MW 683.16, Fig. 7b ). At the end of the reaction, no metalloporphyrin species could be observed owing to the destruction of the metalloporphyrin in the presence of excess ArIO [52] . For [Mn(TDCPP)Cl], the peak at m/z 1283 ([Mn(TDCPP)(ArIO)] + , MW 1283.40) and 1000 ([Mn(O)(TDCPP)(CH 3 CN)] + , MW 1000.27) appeared simultaneously at 15 s ( Fig. 7d ). Later, the ArIO-metalloporphyrin adduct could not be observed when the relative intensity of the peak at 1,000 increased ( Fig. 7e ). Two minutes later after the oxidant was added, the peak at 1,000 reached the maximum while the peak at 1,283 disappeared ( Fig. 7f ), which indicated that the metalloporphyrin-ArIO adduct was completely converted to high valent manganese-oxo species. These results were highly coincident with the ultraviolet–vis spectroscopies (compare Supplementary Fig. S12 and Fig. 7a–c for [Mn(TPP)Cl], Fig. 4a and Fig. 7d–f for [Mn(TDCPP)Cl]). 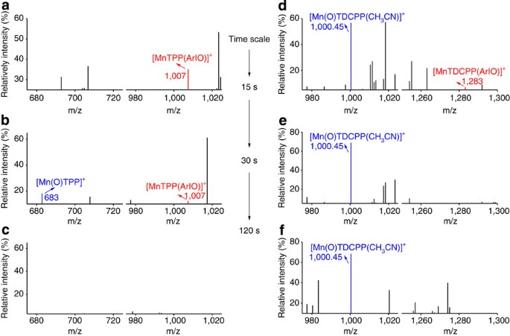Figure 7: ESI-MS analysis of the reaction between manganese porphyrin and ArIO at 15, 30 and 120 s, respectively. ForFig. 7a–c, [Mn(TPP)Cl] was used. ForFig. 7d–f, [Mn(TDCPP)Cl] was used. Figure 7: ESI-MS analysis of the reaction between manganese porphyrin and ArIO at 15, 30 and 120 s, respectively. For Fig. 7a–c , [Mn(TPP)Cl] was used. For Fig. 7d–f , [Mn(TDCPP)Cl] was used. Full size image Therefore, based on the ultraviolet–vis spectroscopies, ESI-MS analysis and kinetic studies, the proposed mechanism shown in Fig. 6 was well supported, and the adducts of Mn(Porphyrins) with ArIO, having the absorption at 460 nm were unambiguously confirmed. In conclusion, by employing soluble iodosylarene 1 as the terminal oxidant, the adducts of iodosylarene with manganese porphyrins as the key intermediate by ultraviolet–vis spectroscopy and ESI-MS analysis were determined in the cytochrome P450 catalysed oxidation from the ‘live’ catalytic oxidative process. When TBPH was used as the reducatnt, the formation of high valent [Mn(por)=O] was the rate-determining step, and ultraviolet–vis spectroscopies of this adduct was characterized. When cis -stilbene was employed as the reductant, co-existence of the adduct and high valent [Mn(Por)=O] were observed. In the absence of reductant, the adduct of iodosylarene with sterically hindered [Mn(TDCPP)Cl] could be immediately formed, and was smoothly converted to the high valent [Mn(Por)=O]. These observations provide preliminary insights toward the mechanism of cytochrome P450. Further mechanistic studies are currently undergoing in our lab, and will be reported in due course. Materials Porphyrins and metalloporphyrins were synthesized by following literature procedures [58] , [59] . Soluble iodosylarene was synthesized from thiophenol as the starting material following Protasiewicz’s method [60] (vide infra). The purity of the oxidant was determined by iodometric titration. TBPH was purchased from Aldrich and recrystallized before use. Cis-stilbene was purchased from Aldrich and used without further purification. CH 2 Cl 2 was dried according to the literature procedures and distilled under N 2 before use. Instrumentation Ultraviolet–vis spectrum was collected on an ultraviolet–vis spectrometer provided from Sinco Corp. (for kinetic study of [Mn(T( p -Cl)PP)Cl], [Mn(T( o -Cl)PP)Cl], [Mn(TDCPP)Cl] and mechanistic study of catalytic reactions and in situ reactions) or an SFM-300 Stopped-Flow purchased from Bio-logic Corp. (for kinetic study of [Mn(TPP)Cl] and [Mn(T( p -OMe)PP)Cl]). GC analysis was obtained from Varian 3900. ESI-MS analysis was obtained from Shimadzu MS 2010ev. Synthesis of tert -butyl(phenyl)sulfane To a 250-ml round bottom flask cooled in an ice bath were successively added acetic acid (20 ml), perchloric acid (70% solution, 7 ml) and acetic anhydride (12 ml) and the solution was stirred for 20 min. Thiophenol (11 g, 50 ml, 100 mmol) and tert -butanol (8.9 g, 11.3 ml, 120 mmol) were added to the mixture and 15 ml of acetic acid was added. The reaction mixture was allowed to warm to room temperature and stirred overnight. The reaction mixture was poured into 100 ml of brine and extracted with diethyl ether (3 × 100 ml). The organic layers were combined, washed with saturated NaHCO 3 aqueous solution (3 × 100 ml), water (100 ml) and dried over Na 2 SO 4 . The solvent was evaporated and the column chromatography of the residue afforded the product as colourless oil (14.02 g, 85%). 1 H NMR (300 MHz, CDCl 3 ) δ 7.52–7.56 (d, J =7.2 Hz, 2 H), 7.32–7.35 (d, J =6.9 Hz, 3 H), 1.29 (s, 9 H). Synthesis of tert -butylsulfonylbenzene Sodium perborate tetrahydrate (27.7 g, 180 mmol) was added to a solution of tert -butyl(phenyl)sulfane (7.5 g, 7.8 ml, 45 mmol) in 100 ml of acetic acid. The cloud suspension was stirred at 50 °C overnight. Acetic acid was removed by reduced pressure distillation, and the residue was poured into 200 ml of water and extracted with diethyl ether (3 × 100 ml). The organic layers were combined, washed with saturated aqueous NaHCO 3 solution (3 × 100 ml) and water (100 ml), and dried over Na 2 SO 4 . The solvent was evaporated and recrystallization of the residue afforded the product as a white solid (8.27 g, 93%). 1 H NMR (300 MHz, CDCl 3 ) δ 7.88 (d, J =7.5 Hz, 2 H), 7.63 (t, J =7.5 Hz, 1 H), 7.56 (t, J =8.1 Hz, 2 H), 1.34 (s, 9 H). Synthesis of 1-( tert -butylsulfonyl)-2-iodobenzene To a solution of tert -butylsulfonylbenzene (8.24 g, 42 mmol) in 50 ml of THF at −78 °C was added 20 ml of n -BuLi in hexane (2.5 M, 50 mmol, 1.2 equiv.) via syringe. After stirring at −78 °C for 40 minutes, a solution of I 2 (12.69 g, 50 mmol, 1.2 equiv.) in 50 ml of THF was added and the reaction mixture was allowed to warm to room temperature and stirred overnight. One hundred milliliter of saturated NH 4 Cl aqueous solution was added to the residue and the organic solvent was removed by evaporation. The mixture was then extracted with diethyl ether (3 × 200 ml). The organic layers were combined, washed with Na 2 SO 3 and dried with MgSO 4 . The solvent was evaporated and recrystallization of the residue afforded the product as a white solid (12.6 g, 93%). 1 H NMR (300 MHz, CDCl 3 ) δ 8.16–8.19 (d, J =7.8 Hz, 1 H), 8.08–8.10 (d, J =7.8 Hz, 1 H), 7.5–7.6 (t, J =6.9 Hz, 1 H), 7.21–7.27 (t, J =6.9 Hz, 1 H), 1.42 (s, 9 H) Synthesis of 1-( tert -butylsulfonyl)-2-iodosylbenzene Sodium perborate tetrahydrate (3.2 g, 21 mmol) was added to a solution of 1-( tert -butylsulfonyl)-2-iodobenzene (650 mg, 2 mmol) in 40 ml of glacial acetic acid at 40–45 °C. The reaction mixture was held at this temperature range and stirred for 5 h. Acetic acid was removed by reduced pressure distillation. The residue was washed with 20 ml water and then extracted with CH 2 Cl 2 (3 × 20 ml). The organic layers were combined, washed with saturated NaHCO 3 aqueous solution until the pH of solution >7, and then dried with Na 2 SO 4 . The solvent was evaporated and recrystallization afforded the product as brilliant yellow solid (524 mg, 77%). 1 H NMR (300 MHz, CDCl 3 ) δ 8.10 (m, 1H), 7.90 (m, 2H), 7.67 (m, 1H), 1.40 (s, 9H). Iodometric titration showed the purity was >95%. Catalytic oxygenation of TBPH An amount of 6.67 × 10 −6 M catalyst MnTPPCl was added into the dichloromethane solution of 1 × 10 −2 M TBPH and 5 × 10 −4 M ArIO at 0 °C. Ultraviolet–vis spectra were collected every 6 s. The baseline was the solvent CH 2 Cl 2 . Monitoring the spectral changes at 477 nm (λ max of [Mn(TPP)Cl] and 630 nm (characteristic absorbance of TBP free radical 4 ) indicated the formation of 4 . For comparison, the reactions were carried out in the absence of MnTPPCl or ArIO. No reactions occurred under these conditions. Catalytic epoxidation of cis -stilbene About 2.5 × 10 −3 M ArIO was added into the CH 2 Cl 2 solution of 1.5 × 10 −2 M cis -stilbene and 6.25 × 10 −6 M [Mn(TPP)Cl] at 0 °C. Ultraviolet–vis spectra were collected every 5 s. The baseline was the mixture combined with cis -stilbene and [Mn(TPP)Cl]. GC analysis showed the formation of cis -stilbene oxide. For comparison, the reactions were carried out in the absence of MnTPPCl or ArIO. No reactions occurred under these conditions. Reaction between ArIO and [Mn(TDCPP)Cl] An amount of 2.5 × 10 −3 M ArIO was added into the CH 2 Cl 2 solution of 6.25 × 10 −6 M [Mn(TDCPP)Cl] at 0 °C in the absence of reductant. Ultraviolet–vis spectra were collected every 5 s. The baseline was the solution of 2e . Two minutes later, 3 was added into the combined solution of 1 and 2e . Reaction between ArI and [Mn(O)(TDCPP)] About 3 × 10 −5 M of ArIO was added into the CH 2 Cl 2 solution of 1 × 10 −5 M [Mn(TDCPP)Cl] at 0 °C in the absence of reductant. One minute later, 4 mg of ArI was added to this mixed solution, and ultraviolet–vis spectra were collected every 2 s. The baseline was the solvent CH 2 Cl 2 . Kinetic measurements All the reactions were performed in CH 2 Cl 2 at 0 °C. Initial rates of the formation of TBP free radical 4 was measured by the increase of the peak at 630 nm (ε=400 M −1 cm −1 ) [32] before the conversion reached to 30%. The concentration of 1 or 3 was maintained as constant while the other one was changed. The rate constants were determined by a least-square curve fit. The first-order plots were linear and all the experiments were performed at least three runs. ESI-MS analysis Four milligram (0.012 mmol, 0.006 M) of oxidant ArIO 1 was dissolved in 2 ml of CH 2 Cl 2 at 0 o C. An amount of 1 × 10 −5 M manganese porphyrin ([Mn(TPP)Cl] or [Mn(TDCPP)Cl]) was injected to this solution. Twenty microliter of this combined solution was taken out and diluted in 2 ml of CH 3 CN for ESI-MS analysis at 15, 30 and 120 s. How to cite this article: Guo, M. et al. Spectroscopic observation of iodosylarene metalloporphyrin adducts and manganese(V)-oxo porphyrin species in a cytochrome P450 analogue. Nat. Commun. 3:1190 doi: 10.1038/ncomms2196 (2012).